5diridium oxide as a material for spin-current detection Devices based on pure spin currents have been attracting increasing attention as key ingredients for low-dissipation electronics. To integrate such spintronics devices into charge-based technologies, electric detection of spin currents is essential. The inverse spin Hall effect converts a spin current into an electric voltage through spin-orbit coupling. Noble metals such as Pt and Pd, and also Cu-based alloys, have been regarded as potential materials for a spin-current injector, owing to the large direct spin Hall effect. Their spin Hall resistivity ρ SH , representing the performance as a detector, is not large enough, however, due mainly because of their low charge resistivity. Here we report that a binary 5 d transition metal oxide, iridium oxide, overcomes the limitations encountered in noble metals and Cu-based alloys and shows a very large ρ SH ~38 μΩ cm at room temperature. Spin-orbit coupling (SOC) is a relativistic effect and relates the spin moment of an electron to its orbital momentum via a momentum-dependent effective magnetic field. In the presence of SOC, a charge current without any spin polarization can be converted into a pure spin current (the flow of spin angular momentum) and vice versa , known as the direct spin Hall effect and the inverse spin Hall effect (ISHE) [1] , [2] , [3] , [4] , [5] , [6] , [7] , [8] , [9] , [10] , [11] , [12] , [13] , [14] , [15] , [16] , [17] , [18] . The presence of these phenomena in non-magnetic semiconductors had already been recognized in 1970s (refs 19 , 20 , 21 , 22 ) but recent theoretical [1] , [2] and experimental investigations [3] , [4] have given a boost to this field. Spin current-based electronics with low-energy consumption has since been discussed, where spin-current injection and detection, using charge/spin conversion by direct spin Hall effect and ISHE, played a key role. A variety of materials have subsequently been explored to realize efficient charge/spin conversion [5] , [6] , [7] , [8] , [9] , [10] , [11] , [12] , [13] , [14] , [15] , [16] , [17] , [18] . The playground for the exploration was first limited to semiconductors but then extended to metals, where we can take advantage of the less pronounced effect of interfacial barriers. Heavy transition metals such as Pt [6] , [7] , [8] , [9] , [10] , [14] , Au [9] , [12] , [13] , and Pd [8] , [9] , [11] and also Cu-based alloys [17] , [18] were found to exhibit a particularly large spin Hall angle α SH (the maximum yield of the charge/spin conversion), 0.01–0.1 at room temperature, owing to their pronounced SOC effects. These effects give these metals an advantage for application as a spin injector. In addition to the large α SH , their low electrical resistivity ( ρ C ), typically ρ C =10 −7 –10 −5 Ω cm, allows large charge currents to be passed and hence to inject a large spin current without serious Joule heating. Spin currents can be detected by using the ISHE. In contrast to the case for spin injectors, the low ρ C of the heavy metals with a large α SH is a disadvantages when it comes to spin detection. In the ISHE, the electric voltage Δ V ISHE generated by a spin current I S is in proportion to ρ C (refs 23 , 24 ): Spin Hall resistivity given by determines the efficiency of spin-current detection. This means that a sensitive detection of spin current could be achieved in materials with both a large α SH and a high ρ C . In typical heavy metals, their low ρ C imposes strong constraints in tuning the value of ρ SH as it remains as low as <1 μΩ cm. One of the obvious approaches to improve the performance of spin detectors could be to increase the ρ C by alloying. Alloying can in fact increase not only the ρ C but also the α SH through an extrinsic spin Hall effect [25] , [26] , [27] . At room temperature where the inelastic scattering of charge carriers is dominant, however, it should be hard to anticipate a drastic increase of ρ C by alloying, for example, more than an order of magnitude increase as compared with the pristine material. Therefore, the improvement of ρ SH would not be achieved only by alloying. In this work, we propose 5 d transition metal oxides (TMOs) as alternative metals to realize both large α SH and large ρ C , which should enhance ρ SH . The uniqueness of 5 d TMOs is characterized by the extremely strong SOC~0.5–1 eV originating from the predominant 5 d character of the conduction band. The SOC in 5 d TMOs is in fact as strong as to reconstruct the electronic structures drastically, as first discussed in the case of J eff =1/2 Mott state Sr 2 IrO 4 (ref. 28 ). The analogous predominant SOC effect has been commonly observed in a broad range of Ir oxides including Ba 2 IrO 4 (ref. 29 ), CaIrO 3 (ref. 30 ) and Ir 2 O 4 (ref. 31 ). In those Ir oxides, in addition to the strong SOC, the localized character of d orbitals gives rise to a moderately high charge resistivity ρ C even in the metallic state. Typical ρ C values of conductive 5 d Ir TMOs such as IrO 2 and SrIrO 3 at room temperature are of the order of 10 −4 –10 −3 Ω cm, at least one order of magnitude higher than those of normal s metals. As the variety of materials continues to grow rapidly, 5 d TMOs offer a unique opportunity to explore the giant ρ SH for efficient spin detection. We selected a simple binary oxide, rutile IrO 2 (refs 32 , 33 , 34 ), as the basis for our exploration. IrO 2 with Ir 4+ shares the same 5 d 5 configuration with many other Ir oxides, where the strong SOC dominates the electronic states and the resultant electronic properties [34] . This binary oxide has been long used as an electrode in various device applications, ranging from non-volatile ferroelectric memories to electrochemical devices. The excellent electrode properties are due to the formation of a clean, well-defined interface with other materials owing to its high chemical and thermal stability, and superior barrier properties for oxygen diffusion. In such a clean interface, it may be possible to inject a spin current through a diffusion process; IrO 2 is therefore an ideal platform for testing the ISHE of 5 d TMOs. Here, we describe successful spin-current injection into IrO 2 using a lateral spin-valve (LSV) device geometry and demonstrate the ISHE with a remarkably high ρ SH as a metal not only in the polycrystalline state but also in the practically important amorphous state. Device structure We fabricated cross-junction-type devices consisting of an IrO 2 wire and a permalloy(Ni 80 Fe 20 , Py)/Ag/Py LSV [35] , shown in Fig. 1a,b (see also Methods). Spin currents are passed in the Ag strip by a non-local charge current injection ( I C ) from the ferromagnetic Py electrode and are perpendicularly injected in part into the IrO 2 wire through the diffusion ( Fig. 1a ). This effect, called spin absorption, enables us to conduct a quantitative analysis of the ISHE as have been demonstrated for various materials [7] , [8] , [17] , [18] . We examined the potential of polycrystalline and amorphous IrO 2 wires as the spin detector element. Their resistivities were 2.0 × 10 −4 Ω cm and 5.7 × 10 −4 Ω cm at 300 K, respectively, which are 1–2 orders of magnitude higher than those of metals that have been studied to date as a spin Hall material. 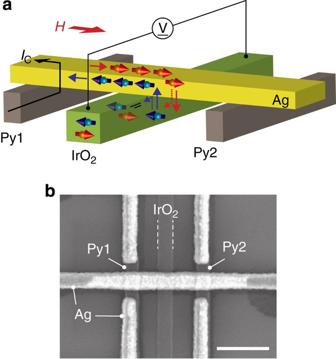Figure 1: Inverse spin Hall effect measurements using a spin absorption effect in a lateral spin-valve geometry. (a) The structure of device used for ISHE measurements is shown schematically. A LSV with two Py electrodes (Py1: spin source, Py2: spin detector) bridged by an Ag spin transport layer was formed on an IrO2wire. Spin-polarized charge current,IC, was injected along the arrow to accumulate pure spin currents in the Ag. The diffusion of spin current into the IrO2wire, namely, the spin absorption, gives rise to the ISHE in IrO2. (b) Scanning electron microscopy image of a typical device. Scale bar, 500 nm. The dotted lines indicate the side edges of the IrO2wire for clarity. Figure 1: Inverse spin Hall effect measurements using a spin absorption effect in a lateral spin-valve geometry. ( a ) The structure of device used for ISHE measurements is shown schematically. A LSV with two Py electrodes (Py1: spin source, Py2: spin detector) bridged by an Ag spin transport layer was formed on an IrO 2 wire. Spin-polarized charge current, I C , was injected along the arrow to accumulate pure spin currents in the Ag. The diffusion of spin current into the IrO 2 wire, namely, the spin absorption, gives rise to the ISHE in IrO 2 . ( b ) Scanning electron microscopy image of a typical device. Scale bar, 500 nm. The dotted lines indicate the side edges of the IrO 2 wire for clarity. Full size image To check that the Ag layer is not oxidized by directly contacting with IrO 2 , we first characterized the Ag/IrO 2 interface by means of interface resistance measurements [36] . The current–voltage characteristics of the Ag/IrO 2 interface showed an ohmic behaviour, typical of metal/metal interface. The slope of the data yielded a resistance–area product (RA) of 2.3 fΩ m 2 at 300 K, which is as low as that of the metallic, transparent Ag/Py interface (RA=1.9 fΩ m 2 at 300 K). An estimate of the thickness of the possibly oxidized Ag layer, using the resistivities of Ag 2 O and AgO in the literature [37] , never exceeded 0.1 nm. These observations imply that the Ag/IrO 2 interface in the present devices is very sharp as in metal/metal interfaces. Spin-current injection into IrO 2 The spin absorption by IrO 2 across the interface was then confirmed by non-local spin-valve (NLSV) experiments [7] , [8] , [17] , [18] , [35] . The schematic diagram of the measurement is shown in Fig. 2a . The pure spin currents accumulated in the Ag strip by injecting spin-polarized charge currents I C from Py1 to Ag is detected as a voltage V S (= V + − V − ) between Py2 ( V + ) and Ag ( V − ) (upper panel). The spin accumulation signal Δ R S is given by the difference in V S / I C ( R S ) between parallel (high R S ) and antiparallel (low R S ) magnetizations of the two Py wires. If an IrO 2 middle wire is in contact with the Ag, the accumulated spin diffuses in part into it (lower panel), resulting in the reduction in Δ R S (ref. 7 ). 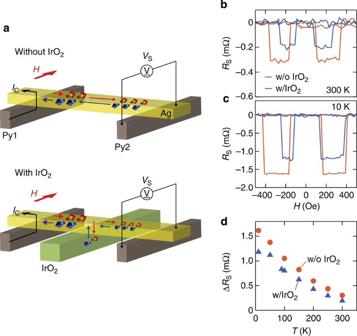Figure 2: Non-local spin-valve measurements. (a) The set-up of measurement is schematically depicted. The magnetic fieldHis applied along the easy axis of the Py electrodes. (b,c) NLSV signals measured at 300 K and 10 K for Py/Ag/Py LSVs without and with the polycrystalline IrO2middle wire. (d) Temperature dependences of the NLSV signals. Figure 2b and c show field dependences of R S at 300 and 10 K, respectively. The decrease of Δ R S by the insertion of the IrO 2 middle wire indicates the spin absorption effect. This is more clearly demonstrated in the t emperature ( T ) dependence of Δ R S with (Δ R S with ) and without (Δ R S without ) the middle wire, as displayed in Fig. 2d . At all the temperatures, Δ R S with is systematically smaller than Δ R S without , while both are enhanced at low temperatures owing to the increase of the spin-diffusion length of Ag ( λ Ag ) [35] . By analysing the data based on the three-dimensional spin-diffusion model [18] (see Supplementary Methods and Supplementary Fig. S1 ), we estimated a spin-diffusion length in polycrystalline IrO 2 , =3.8 nm at 300 K and 8.4 nm at 10 K, which are comparable to those of Pt (3–10 nm at 300 K (refs 6 , 7 , 8 , 9 , 10 , 14 )) and CuIr (5–20 nm at 10 K (ref. 17 )) where relatively large spin Hall angles were observed. This indicates that spin scattering of IrO 2 is indeed very strong as expected from the 5 d conduction band [34] . Figure 2: Non-local spin-valve measurements. ( a ) The set-up of measurement is schematically depicted. The magnetic field H is applied along the easy axis of the Py electrodes. ( b , c ) NLSV signals measured at 300 K and 10 K for Py/Ag/Py LSVs without and with the polycrystalline IrO 2 middle wire. ( d ) Temperature dependences of the NLSV signals. Full size image ISHE and ρ SH of IrO 2 By injecting spin currents through the spin absorption effect, we successfully observed ISHE in IrO 2 . In Fig. 3a,b , we plot the room-temperature ISHE signal R ISHE (≡Δ V ISHE / I C ) for polycrystalline and amorphous samples as a function of the magnetic field (The temperature dependence of the ISHE is shown in Supplementary Fig. S2 and is explained in Supplementary Note 1 ). Here the magnetic field was applied along the hard axis of the Py spin source (see Fig. 1a ), and Δ V ISHE was induced along the long-axis direction of the IrO 2 wire. Reflecting the magnetization process in hard axis of Py, R ISHE linearly increased up to ~1,500 Oe and then saturated. The antisymmetric response to the applied magnetic field excludes any spurious effects such as anisotropic magnetoresistance of Py; the ISHE of IrO 2 is responsible for the resistance change (2Δ R ISHE ) between positive and negative magnetic fields. The in-plane angular dependence of magnetic field effect on R ISHE was confirmed fully consistent with the ISHE origin. 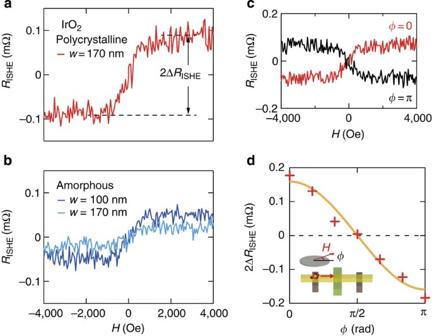Figure 3: Inverse spin Hall effect of IrO2at 300 K. (a) The ISHE signalRISHE(≡ΔVISHE/IC) for a polycrystalline IrO2wire with a widthwof 170 nm was measured as a function of the applied magnetic fieldH. (b) The results for amorphous IrO2samples. Two devices with differentwvalues (100 and 170 nm) were measured. The 100 nm-width device showed largerRISHEbecause of the increase of spin-current density.RISHEof the two amorphous devices are smaller than that of the polycrystalline sample shown ina. (c,d) Angular dependence ofRISHEand the resistance change 2ΔRISHEby the ISHE. The in-plane azimuthal angleφwith respect to the long axis of Ag is rotated to change the polarization direction of the spin current (inset ind). The solid line indis a cosφcurve fitted to the results. Figure 3c shows the variation in R ISHE under a magnetic field direction rotated by φ with respect to the ordinary set-up ( Fig. 3d , inset). The sign change of R ISHE occurs between φ =0 and π by magnetization switching of Py and concomitant polarization reversal of the spin current. As shown in Fig. 3d , the resistance change 2Δ R ISHE vanishes at φ = π /2 and exhibits a cos φ relation. This characteristic angular dependence is the hallmark of ISHE [7] , [12] , evidencing spin-dependent electron scattering in IrO 2 . Figure 3: Inverse spin Hall effect of IrO 2 at 300 K. ( a ) The ISHE signal R ISHE (≡Δ V ISHE / I C ) for a polycrystalline IrO 2 wire with a width w of 170 nm was measured as a function of the applied magnetic field H . ( b ) The results for amorphous IrO 2 samples. Two devices with different w values (100 and 170 nm) were measured. The 100 nm-width device showed larger R ISHE because of the increase of spin-current density. R ISHE of the two amorphous devices are smaller than that of the polycrystalline sample shown in a . ( c , d ) Angular dependence of R ISHE and the resistance change 2Δ R ISHE by the ISHE. The in-plane azimuthal angle φ with respect to the long axis of Ag is rotated to change the polarization direction of the spin current (inset in d ). The solid line in d is a cos φ curve fitted to the results. Full size image Because of the large difference in ρ C between Ag and IrO 2 , the charge current induced in the IrO 2 wire by the ISHE is partially shunted by the adjacent Ag layer. To take into account such geometric effects and to precisely determine ρ SH , we adopted the three-dimensional spin-diffusion model (see also Supplementary Methods ). 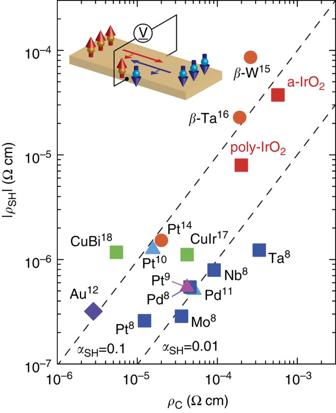Figure 4: Spin Hall resistivity of metals. Experimentally measured values of spin Hall resistivityρSHfor various metals are plotted as a function of electrical resistivityρC. Data include Pt (refs9,10) and Pd (ref.11) evaluated at room temperature by spin pumping, Pt (ref.14) and atomic layer thin films of β-W (ref.15) and β-Ta (ref.16) at room temperature by spin-transfer-torque ferromagnetic resonance, Au at 295 K using a planar Hall device12, Ta, Nb, Pd, Mo, Pt (ref.8), 12% Ir-doped Cu (ref.17), 0.5% Bi-doped Cu (ref.18) at 10 K, and polycrystalline and amorphous IrO2at 300 K (this work) by spin absorption. Using the ISHE signal 2Δ R ISHE and data obtained from the NLSV measurements, α SH and ρ SH are, respectively, calculated to be 0.040 and 8.0 μΩ cm for polycrystalline IrO 2, and 0.065 and 37.5 μΩ cm for amorphous IrO 2 at 300 K. Figure 4 summarizes spin Hall resistivity ρ SH and electrical resistivity ρ C for a variety of metals with a large spin Hall angle α SH reported so far, together with that for IrO 2 . It mimics the point of this work in that ρ SH of IrO 2 is distinctly large compared with typical heavy metals and their alloys of which ρ SH is ~0.16–1.2 μΩ cm (refs 6 , 7 , 8 , 9 , 10 , 11 , 12 , 13 , 14 , 17 , 18 ), and is now comparable to the large ρ SH that was recently discovered in ultrathin films of β-phase (A15 crystal structure) W (ref. 15 ) and Ta (ref. 16 ). Figure 4: Spin Hall resistivity of metals. Experimentally measured values of spin Hall resistivity ρ SH for various metals are plotted as a function of electrical resistivity ρ C . Data include Pt (refs 9 , 10 ) and Pd (ref. 11 ) evaluated at room temperature by spin pumping, Pt (ref. 14 ) and atomic layer thin films of β-W (ref. 15 ) and β-Ta (ref. 16 ) at room temperature by spin-transfer-torque ferromagnetic resonance, Au at 295 K using a planar Hall device [12] , Ta, Nb, Pd, Mo, Pt (ref. 8 ), 12% Ir-doped Cu (ref. 17 ), 0.5% Bi-doped Cu (ref. 18 ) at 10 K, and polycrystalline and amorphous IrO 2 at 300 K (this work) by spin absorption. Full size image To generate a large electric voltage using the ISHE of IrO 2 from existing metal-based spin-current devices, it is important to reduce the shunting effect at the Ag/IrO 2 interface due to their large difference in ρ C . One of the promising approaches is to use Al (ref. 38 ) and Mg (ref. 39 ) as the non-magnetic spin transport layer. Their ρ C values are one order of magnitude higher than that of Ag we used, of the order of 10 μΩ cm at room temperature, while a comparably long spin-diffusion length is obtained. Another interesting route is a spin transport layer based on a conductive oxide composed of light elements with small SOC. For example, in ZnO (ref. 40 ), doping with Al yields ρ C of the order of 100 μΩ cm (ref. 41 ), which can match with that of IrO 2 . The high chemical stability of IrO 2 could be advantageous in fabricating such oxide-based junctions. The discovery of the ISHE in amorphous IrO 2 , which can be grown at room temperature, is a significant step towards spintronics devices based on such oxide materials. The comparably large α SH in the amorphous form may point to that spin scattering in this compound occurs at the length scale of as short as a unit cell, potentially enabling the spin detection at the atomic layer thickness. Although the physics of spin scattering in amorphous states has not been understood yet, the availability of the amorphous form should make it easier to study SOC-induced transport phenomena in 5 d TMOs not used before in spintronics. In conclusion, 5 d TMOs are the most promising materials for spin detection in spintronics. We demonstrated that the combination of strong SOC and a moderately high ρ C is a key to improve the performance of spin detection. These achievements in the simple binary oxide manifest the potential of 5 d TMOs as a new class of spintronic materials. Strong SOC in this class of materials produces a rich variety of intriguing physical properties, including correlated topological insulator [42] , Weyl semi-metal [43] and Kitaev spin liquid [44] . Our discovery of the large spin Hall resistivity may make 5 d TMOs even more fascinating. Device fabrication The Py/Ag/Py LSV with an IrO 2 middle wire was fabricated on a SiO 2 /Si substrate. Au/Ti leads for electrical measurements were prepared on the substrate by a photolithography and an e-beam deposition. IrO 2 film was grown by a reactive sputtering with a 99.9% pure Ir target. A wire structure of IrO 2 was formed using a posi-type resist patterned by an e-beam lithography. The typical wire width and thickness were 170 and 15 nm, respectively. During the deposition, the substrate was not heated, and the pressure was fixed at 0.7 Pa of Ar/O 2 (90:10) mixture gas. X-ray diffraction analysis indicated that the as-deposited IrO 2 film was amorphous. The amorphous film turned into polycrystalline after a post-annealing at 400 °C in air. The LSV with a Py–Py separation of 700 nm (centre-to-centre) was then formed onto the IrO 2 wire by the shadow evaporation method [35] , [36] . To prevent the surface oxidation of Ag, a 2-nm-thick MgO protection layer was e-beam deposited on the surface without breaking vacuum. The width and thickness of wire were 170 and 100 nm for Ag, and 170 and 20 nm for Py, respectively. Their ρ C and spin-diffusion length were 3.0 μΩ cm and 330 nm for Ag and 47 μΩ cm and 5 nm for Py, respectively, at 300 K. One of the two Py electrodes was made longer than the other (not shown in Fig. 1b ) to make the contrast in the fields for magnetization reversal. Electrical measurements All electrical measurements were performed by a standard lock-in technique in a He flow cryostat. An alternating current I C of 200 μA with a frequency of 79 Hz was used for NLSV measurements. In ISHE measurements, I C of 400 μA was applied. We confirmed the linearity between the output voltage Δ V ISHE and I C in the range of 100–400 μA. How to cite this article: Fujiwara, K. et al. 5 d iridium oxide as a material for spin-current detection. Nat. Commun. 4:2893 doi: 10.1038/ncomms3893 (2013).